Control of membrane gaps by synaptotagmin-Ca2+measured with a novel membrane distance ruler Fast synchronous neurotransmitter release is triggered by calcium that activates synaptotagmin-1 (syt-1), resulting in fusion of synaptic vesicles with the presynaptic membrane. Syt-1 possesses two Ca 2+ -binding C2 domains that tether membranes via interactions with anionic phospholipids. It is capable of crosslinking membranes and has recently been speculated to trigger fusion by decreasing the gap between them. As quantitative information on membrane gaps is key to understanding general cellular mechanisms, including the role of syt-1, we developed a fluorescence-lifetime based inter-membrane distance ruler using membrane-anchored DNAs of various lengths as calibration standards. Wild-type and mutant data provide evidence that full-length syt-1 indeed regulates membrane gaps: without Ca 2+ , syt-1 maintains membranes at distances of ~7–8 nm. Activation with 100 μM Ca 2+ decreases the distance to ~5 nm by binding the C2 domains to opposing membranes, respectively. These values reveal that activated syt-1 adjusts membrane distances to the level that promotes SNARE complex assembly. Neurotransmission is accomplished by exocytosis following the fusion of synaptic vesicles with the presynaptic plasma membrane [1] , [2] , [3] . The neurotransmitters stored within the vesicles are released into the synaptic cleft at a millisecond timescale on Ca 2+ influx [4] , with syt-1, residing on the synaptic vesicles and bearing two Ca 2+ -binding C2 domains (C2A and C2B), being the indispensable Ca 2+ sensor [5] , [6] ( Fig. 1 ). The C2A and C2B domains, after coordinating to multiple Ca 2+ ions [7] , [8] , [9] , bind to membranes containing negatively charged phospholipids, which complete the Ca 2+ -coordination sites [8] . Moreover, a patch of four lysine residues (KKKK, 324–327) located on the side of C2B interacts specifically with the poly-anionic phosphatidylinositol(4,5)-bisphosphate (PIP2) in a Ca 2+ -independent manner [10] . However, despite extensive research using either the full-length syt-1 (including the transmembrane domain, TMD) or the truncated soluble C2AB fragment [11] , [12] , [13] , the questions how syt-1 functions at a molecular level as a Ca 2+ -trigger and how it interacts with the SNARE proteins (soluble N -ethylmaleimide-sensitive factor attachment protein receptor), the membrane fusion machinery [1] , [2] , remained unsettled. 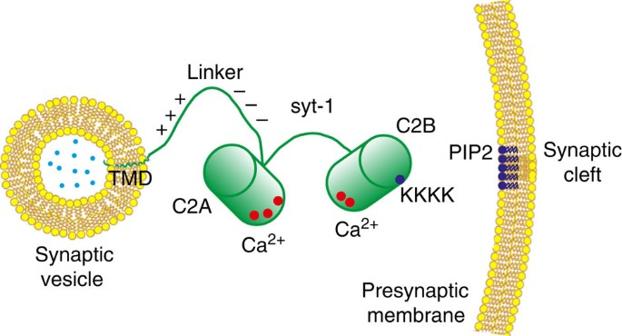Figure 1: Schematic illustration of the synaptotagmin-1 domain structure. Red dots indicate Ca2+-binding sites of the two Ca2+-binding domains C2A and C2B, whereas the dark blue dot represents the poly-lysine patch (KKKK) of the C2B domain. Plus and minus signs indicate clusters of positive and negative charges on the linker. Bright blue dots represent neurotransmitter molecules. PIP2, phosphatidylinositol(4,5)-bisphosphate; TMD, transmembrane domain. Figure 1: Schematic illustration of the synaptotagmin-1 domain structure. Red dots indicate Ca 2+ -binding sites of the two Ca 2+ -binding domains C2A and C2B, whereas the dark blue dot represents the poly-lysine patch (KKKK) of the C2B domain. Plus and minus signs indicate clusters of positive and negative charges on the linker. Bright blue dots represent neurotransmitter molecules. PIP2, phosphatidylinositol(4,5)-bisphosphate; TMD, transmembrane domain. Full size image Before the formation of fully zippered SNARE complexes, which exert forces on the membranes and lead consequently to fusion, the synaptic vesicles are first primed to the presynaptic plasma membrane and await the Ca 2+ activation of syt-1. The models describing the molecular activation of the fusion reaction by synaptotagmin fall into two groups (summarized in ref. 14 ). In the first scenario, the SNARE complexes are arrested at a partially zippered state during the priming process. Syt-1 may either serve as a fusion clamp that is released on Ca 2+ triggering [15] , or alternatively, it may displace the inhibitory protein complexin from the SNARE complexes [16] . In the second scenario, the SNAREs do not assemble before arrival of the Ca 2+ signal, although syt-1 may already be in contact with the plasma membrane via the KKKK–PIP2 electrostatic interaction [10] . Following Ca 2+ triggering, the SNAREs rapidly progress through zippering and fusion [17] . In line with the latter scenario, recently, it has been proposed that syt-1 triggering is based on Ca 2+ -dependent regulation of the gap between the vesicle and presynaptic membranes. In the absence of Ca 2+ , syt-1 connects membranes via (i) its own transmembrane domain and (ii) binding to PIP2 via the KKKK polybasic stretch. Assuming that the 61-residue linker [18] between C2A and the transmembrane domain is unstructured and stretched, a maximal distance of ~28 nm is feasible. On the basis of non-quantitative Förster resonance energy transfer (FRET) between labelled lipids in the participating membranes, it was suggested that addition of Ca 2+ might reduce the distance to a range of ~2–7.5 nm (ref. 19 ). Such distance shortening might operate upstream of the SNARE complex formation, which requires a membrane distance below 8 nm (ref. 20 ). However, experimental support for this model was still elusive, primarily because of the lack of experimental evidence for distance variations at the appropriate length scale. In this study, we first developed a quantitative membrane distance assay based on accurate fluorescence lifetime detection of multiple inter-membrane FRET interactions between tethered small unilamellar liposomes using membrane-anchored double-stranded DNA (dsDNA) of defined lengths as calibration standards. This calibrated system was then used to measure membrane distances of liposomes tethered by full-length syt-1 wild-type as well as Ca 2+ -binding mutants in the absence and presence of physiological Ca 2+ concentrations and when the content of anionic lipids required for syt-1 binding was varied. These data provide evidence that Ca 2+ -activated syt-1 indeed decreases membrane gaps to a level of ~5 nm, which corresponds to the inter-membrane distance spanned by a trans- SNARE complex. Membrane distance ruler The fluorescence lifetime of donor molecules labelled on lipid headgroups (Oregon Green 488 DHPE) of the DNA- or proteoliposomes was chosen as a robust indicator of FRET, as it is insensitive to variations in the concentration of liposomes within the confocal volume of ~1 femtoliter or to variations in alignment conditions of the experimental set-up. In contrast to FRET-based distance measurements within or between interacting proteins [21] , [22] , [23] , distances between membranes cannot be easily extracted. In proteins, single donor and acceptor dyes are attached to defined sites and a single donor–acceptor pair is distant from the other fluorophores. In these cases, the average distance between the pair can be easily derived, providing that the Förster distance R 0 for the selected donor and acceptor is known. On liposomes, contrarily, the fluorophores are distributed across the surfaces of both the inner and outer leaflets. Hence, in a single tethered cluster, each donor molecule may transfer the excitation energy to multiple acceptors, and the probability of each donor undergoing FRET is different and depends on its position relative to the acceptor liposomes containing Texas Red DHPE ( Fig. 2a ), which in turn leads to different lifetimes. Therefore, we measured first a calibration curve using tethered liposomes with predefined spacings so that the average donor fluorescence lifetimes can be correlated properly with membrane distances between donor and acceptor liposomes. The calibration of this membrane distance ruler was done using membrane-anchored dsDNA of various well-defined lengths as discrete spacers [24] . In general, dsDNA shorter than its persistence length of 50 nm, or 150 base pairs (bp), is known to have high bending rigidity [25] . Herein three different lengths well below the persistence length were prepared ( Fig. 2 ), 3.3 nm (10 bp), 5.0 nm (15 bp) and 8.3 nm (25bp). The membrane anchor lipid 1,2- O -dioctadecyl-(rac)-glycerol was attached to the 5′-end of DNA oligonucleotides by solid-phase synthesis using a synthetic lipid phosphoramidite [26] . The complementary strands were then individually reconstituted into the donor and acceptor liposomes, respectively. In addition, 10% anionic lipids phosphatidylserine (PS) were included in both types of DNA liposomes. The negative charges on the liposome surfaces and the negatively charged DNA backbone further stabilized the perpendicular orientation of the DNA already observed in the absence of any repulsive charges on the membranes [27] . 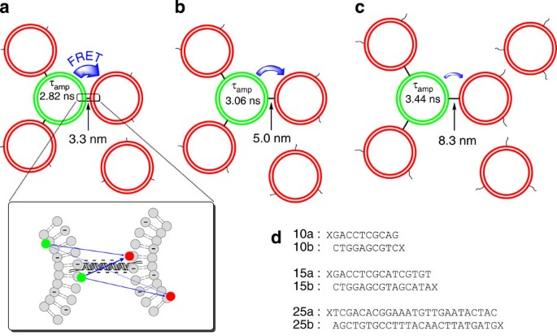Figure 2: FRET from green donor liposomes to the surrounding red acceptor liposomes. The upper panels show the experimental design of the membrane distance ruler for small unilamellar liposomes, with (a) 3.3, (b) 5.0 and (c) 8.3 nm spacings. FRET decreases as the distance increases, as reflected in the longer amplitude-weighted lifetime (τamp). (d) The complementary DNA sequences for the respective lengths, where X denotes the lipid-phosphoramidite. Figure 2: FRET from green donor liposomes to the surrounding red acceptor liposomes. The upper panels show the experimental design of the membrane distance ruler for small unilamellar liposomes, with ( a ) 3.3, ( b ) 5.0 and ( c ) 8.3 nm spacings. FRET decreases as the distance increases, as reflected in the longer amplitude-weighted lifetime ( τ amp ). ( d ) The complementary DNA sequences for the respective lengths, where X denotes the lipid-phosphoramidite. Full size image An excess of acceptor liposomes was used to drive the equilibrium so that each donor liposome is surrounded by an equal (maximal) number of acceptor liposomes ( Fig. 2a–c ), to eliminate the contribution of differences in the degree of tethering [28] . To determine the required ratio, we gradually increased the acceptor liposome concentration while keeping the donor liposomes constant. The donor fluorescence decay curves converged after the ratio exceeded 1:10 ( Supplementary Fig. 1 ). Therefore, a ratio of 20 acceptor liposomes to 1 donor liposome was selected for all experiments. The fluorescence decay curves of the three DNA-tethered liposome mixtures were measured with time-correlated single photon counting [29] (TCSPC) ( Fig. 3a ), and the emission wavelength was selected at the blue edge of donor fluorescence spectrum (525±10 nm) to minimize the crosstalk between donor and acceptor channels ( Supplementary Fig. 2 ). The three curves were clearly distinguishable and decayed faster than the control sample without DNA, and the difference arises predominantly from the donor molecules that are facing the acceptor liposomes. The decay curves observed with the aforementioned excess ratio of 1:20 were fitted with two components, and the amplitude-weighted lifetimes ( τ amp , see Methods section) of the donors depending on inter-membrane distances were obtained. By measuring three independent replicates, τ amp for liposomes with membrane distances of 8.3, 5.0 and 3.3 nm was determined to be 3.44±0.05, 3.06±0.13 and 2.82±0.18 ns, respectively (average±s.d.). A plot of τ amp versus the membrane distance can be very well fitted by a linear approximation ( Fig. 3g ), which later serves as the calibration curve for membrane distance determination. As control, hybridization of complementary DNA strands on the liposomes was inhibited by adding a free single strand (without the lipid anchor, Supplementary Fig. 3 ). Under these conditions, the lifetime was restored to the control level observed with a sample containing donor and excess acceptor liposomes, neither with DNA. An advantage of the calibration procedure ( Fig. 3g ) is that any nonspecific effects, such as nonspecific liposome clustering, are intrinsically corrected for. To quantify the extent of such nonspecific effects, we compared a sample containing only pure donor liposomes (grey dashed line in Supplementary Fig. 3 ) directly with the donor–acceptor control without any DNA (black line in Supplementary Fig. 3 ). This comparison demonstrates that nonspecific effects contribute only to a minor extent to the overall fluorescence decay. 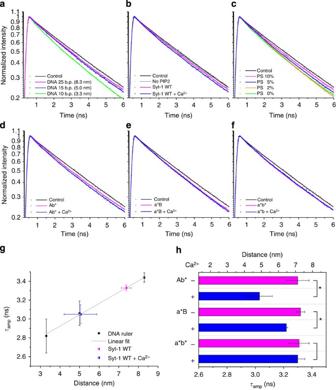Figure 3: The measured fluorescence decay curves and the membrane distance ruler for converting fittedτampinto closest distances between small unilamellar liposomes. Decay curves for (a) DNA-tethered liposomes with specified number of base pairs and (b) syt-1 wild-type (WT) reconstituted into donor liposomes in the absence and presence of 100 μM Ca2+. No PIP2 indicates the sample in which 2% PIP2 was substituted with 7% PS. (c) Measurements without Ca2+for syt-1 WT reconstituted into donor liposomes with various molar ratios of the anionic lipid PS. (d–f) Decay curves for Ab*, a*B and a*b* mutants. Control stands for the experiments in which there was no protein or DNA on either type of liposomes. The symbols represent experimental data, whereas the lines are reconvolution fits using two exponentials. (g) The plot of amplitude-weighted lifetime (τamp) versus distance. A linear regression line can be constructed with the DNA-tethered liposomes and applied to determine the distance between syt-1 tethered liposomes in the absence or presence of 100 μM Ca2+. (h)τampand the calculated distance information for the mutants. The error bars represent s.d. values obtained from three independent repeats. Asterisks (*) designate when theτampvalues are statistically different (P<0.05, two-tailed unpairedt-test). Figure 3: The measured fluorescence decay curves and the membrane distance ruler for converting fitted τ amp into closest distances between small unilamellar liposomes. Decay curves for ( a ) DNA-tethered liposomes with specified number of base pairs and ( b ) syt-1 wild-type (WT) reconstituted into donor liposomes in the absence and presence of 100 μM Ca 2+ . No PIP2 indicates the sample in which 2% PIP2 was substituted with 7% PS. ( c ) Measurements without Ca 2+ for syt-1 WT reconstituted into donor liposomes with various molar ratios of the anionic lipid PS. ( d – f ) Decay curves for Ab*, a*B and a*b* mutants. Control stands for the experiments in which there was no protein or DNA on either type of liposomes. The symbols represent experimental data, whereas the lines are reconvolution fits using two exponentials. ( g ) The plot of amplitude-weighted lifetime ( τ amp ) versus distance. A linear regression line can be constructed with the DNA-tethered liposomes and applied to determine the distance between syt-1 tethered liposomes in the absence or presence of 100 μM Ca 2+ . ( h ) τ amp and the calculated distance information for the mutants. The error bars represent s.d. values obtained from three independent repeats. Asterisks (*) designate when the τ amp values are statistically different ( P <0.05, two-tailed unpaired t -test). Full size image It is known from electron microscopy (EM) studies that small unilamellar liposomes (≤50 nm), owing to their high membrane curvature, still maintain the spherical shape at contact areas when tethered by proteins (see for example, cryo-electron tomography in ref. 30 ). To ensure additionally that the number of membrane tethering sites between donor and acceptor liposomes are comparable in all samples, we conducted fluorescence correlation spectroscopy (FCS, see Supplementary Fig. 4 and Supplementary Methods for details). FCS data showed that the average number of acceptor liposome tethering sites per donor liposome did not vary by >15% throughout all samples measured in this work ( Supplementary Table 1 ). Synaptotagmin-1 controls the gap between two membranes Next, we reconstituted syt-1 in donor liposomes containing 10% PS and measured the decay when they were bound to acceptor liposomes bearing 15% PS plus 2% PIP2 ( Fig. 3b ) [3] , [31] . In the absence of Ca 2+ (1 mM EGTA), τ amp was close to that of the 8.3 nm DNA-tethered liposomes (3.33±0.03 ns) and the membrane distance was estimated to be 7.4 nm ( Fig. 3b,g ). To verify that the decrease in fluorescence lifetime compared with the control sample was caused by the specific interaction of the KKKK patch with PIP2, the poly-anionic PIP2 (2%) in the acceptor liposomes was replaced by increasing the concentration of mono-anionic PS by 7 to 22% PS, which maintained the net negative charge of the acceptor liposomes [32] . In the absence of PIP2, the fluorescence lifetime returned to the control level, showing that tethering to the syt-1 proteoliposomes was abolished. We then repeated the incubation using PIP2-containing liposomes in the absence of Ca 2+ (1 mM EGTA) to allow for the KKKK-PIP2 binding and added appropriate Ca 2+ buffer afterwards to achieve a final free Ca 2+ concentration of 100 μM. The resulting fluorescence decay was accelerated and corresponded to that measured with liposomes tethered with the DNA-ruler at a distance of 5.0 nm ( τ amp =3.05±0.10) ( Fig. 3b,g ). We conclude accordingly that the gap between syt-1 proteoliposomes and the surrounding acceptor liposomes decreases to ~5 nm after the addition of Ca 2+ . The distance of 7.4 nm in the absence of Ca 2+ is relatively short, suggesting that the linker between the transmembrane domain and the C2A domain is not completely stretched [19] . Intriguingly, the linker contains a membrane-adjacent stretch of positive charges, which may interact with the more C-terminally localized stretch of negative charges [33] and/or with anionic lipids in the resident membrane of the protein (a cis interaction) [34] . To further examine the electrostatic interactions with negative charges on the liposome membranes [28] , we performed a set of experiments in which the content of PS on the donor proteoliposomes was varied ( Fig. 3c ). When the donor proteoliposomes were neutral, that is, without PS, and only the acceptor liposomes contained anionic lipids, the measured lifetime was surprisingly short (2.82±0.09 ns) even in the absence of Ca 2+ and was similar to that of the shortest set of DNA-tethered liposomes (3.3 nm). This short distance can be explained by the nonphysiological elimination of electrostatic repulsion between the two membranes, which is present in vivo between the negatively charged synaptic vesicle and presynaptic membranes [3] , [31] . In addition, the membranes may be pulled into close proximity if the positively charged lysine residues on the linker are attached in trans to the surfaces of acceptor liposomes. Figure 3c also indicates that at an intermediate level of PS (5%), there is an equilibrium between the 7.4- and 3.3-nm configurations. Ca 2+ -binding mutants As all known Ca 2+ effects are mediated by the Ca 2+ -binding sites in the C2A and C2B domains, we repeated the distance measurements using previously characterized syt-1 mutants in which Ca 2+ binding to the C2A, C2B or to both C2 domains was disrupted (a*B: D178A, D230A and D232A; Ab*: D309A, D363A and D365A; a*b*: D178A, D230A, D232A, D309A, D363A and D365A) [11] . In the mutant with a disrupted C2B domain (Ab*), the inter-membrane distances in the absence and presence of Ca 2+ were very similar to those of the wild-type protein ( Fig. 3d,g,h ). In contrast, in the mutants with a disrupted C2A domain (a*B and a*b*), there was little or no distance shortening on addition of Ca 2+ , respectively ( Fig. 3e,f,h ). Summarized in Fig. 3h are the fitted τ amp and the corresponding distances calculated for all mutants. These data support a model according to which the C2A domain is predominantly responsible for distance shortening due to Ca 2+ -mediated cis binding to its own membrane. On the contrary, the C2B domain, at least under our experimental conditions, does not appear to be capable of simultaneous cis - trans binding as previously suggested [8] , [35] . The fact that a*B still exhibits a minor decrease in distance on Ca 2+ addition may rather be explained by the Ca 2+ -induced binding of C2B to the acceptor membrane and the insertion of its hydrophobic residues [10] , [36] . The calibrated fluorescence-lifetime-based membrane distance ruler with membrane-anchored DNAs of well-defined lengths allowed for direct quantitative determination of membrane gaps controlled by wild-type and mutants of the full-length neurotransmission trigger syt-1. Initially, in the absence of Ca 2+ , the poly-lysine patch (KKKK) located on the C2B domain is targeted to PIP2 clusters on the presynaptic plasma membrane ( Fig. 4a,b ) [37] , [38] . Our data demonstrate that at this stage full-length syt-1 maintains the two membrane bilayers at a distance of ~7–8 nm ( Fig. 4b ), which is much shorter than a maximum length of ~28 nm if the linker would be unstructured and fully stretched. The ~7–8 nm distance corresponds to that when the SNARE motifs start to assemble and form the coiled coil four-helix bundle (measured with surface forces apparatus) [20] , implying that syt-1 holds the two membranes at this distance so that the fusion machinery is ready for fast initiation [17] . Recently, such a pre-triggered state was also captured in cryo-EM images in ref. 30 , which revealed that a large number of small liposomes incorporating syt-1 and synaptobrevin (the vesicle -SNARE protein) remained docked to giant liposomes including syntaxin and SNAP-25 (the target -SNAREs) at distances on the order of ~10 nm, even after extended incubation. The fact that removing synaptobrevin or adding its soluble counterpart to inhibit the full-length SNARE assembly did not alter the overall tethering suggests the major role of syt-1 in establishing a first contact to the target membrane, upstream of SNARE nucleation ( Fig. 4b ) [19] , [39] . 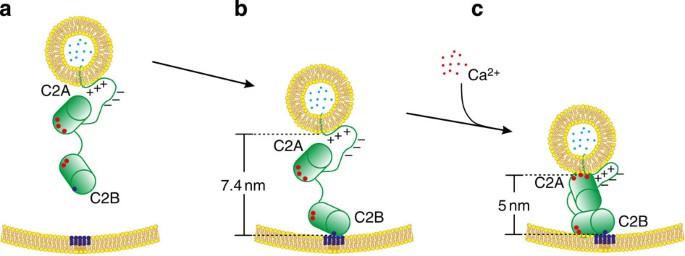Figure 4: Model of full-length syt-1 binding across the synaptic vesicle and the presynaptic plasma membrane. (a) Syt-1 targets PIP2 clusters via the poly-lysine patch (blue). (b) The distance between two membranes is maintained at ~7-8 nm, as the linker is not fully stretched34. (c) On Ca2+influx, the C2A domain bindscis, reducing the distance to 5 nm and potentially promoting the electrostatic zippering of the linker33. Both membranes contain PS. Figure 4: Model of full-length syt-1 binding across the synaptic vesicle and the presynaptic plasma membrane. ( a ) Syt-1 targets PIP2 clusters via the poly-lysine patch (blue). ( b ) The distance between two membranes is maintained at ~7-8 nm, as the linker is not fully stretched [34] . ( c ) On Ca 2+ influx, the C2A domain binds cis , reducing the distance to 5 nm and potentially promoting the electrostatic zippering of the linker [33] . Both membranes contain PS. Full size image Second, the ruler provides clear evidence that, on Ca 2+ influx, the inter-membrane gap is compressed to ~5 nm ( Fig. 4c ). As a trans- SNARE complex spans two membranes at a distance of ≥4 nm (ref. 40 ), a distance reduction from ~7–8 nm to ~5 nm brings the two membranes to a level at which very likely full assembly of the SNAREs is promoted [41] , leading subsequently to the initiation of membrane fusion and neurotransmitter release. At first glance, the ~2.4 nm change in distance may not seem very large in terms of the absolute value. However, considering the above-mentioned dimensions of the SNAREs, such a change is quite significant and allows for efficient triggering at the millisecond timescale. The membrane distance of 5 nm also correlates to cryo-EM observations [35] , [42] for liposomes clustered by soluble C2AB fragments incorporating Ca 2+ , in which the C2A and C2B domains bind to opposing membranes [43] . Such an antiparallel conformation has been shown to be of the lowest energy from simulated annealing based on EPR-derived restraints using the soluble C2AB fragment [44] , [45] , [46] . Moreover, it corroborates new findings that alteration in the length and rigidity of the short (9-residue) linker between the C2 domains has a significant impact on evoked neurotransmitter release [47] . In vivo mutation studies demonstrated that the C2B domain is indispensable for fast synchronous neurotransmitter release [48] , [49] . The fact that the distance regulation behaviour of the Ab* mutant is similar to that of the wild-type ( Fig. 3g,h ) illustrates that in contrast to the C2B domain—which plays an essential general role—C2A plays a more important role in the distance regulation itself: initially, the C2B domain is needed to tether the membranes together, especially via its poly-lysine patch also in the absence of Ca 2+ ( Fig. 4b ). After C2B is already attached to the opposite membrane, an effective decrease of the inter-membrane gap can then be accomplished by binding of the C2A domain back to the host membrane and an even tighter binding of the C2B domain to the opposite membrane with Ca 2+ coordination ( Fig. 4c ). Obviously, the role of C2B Ca 2+ binding sites is less connected to the distance regulation function of syt-1 than to other important mechanistic functions, which might include direct interactions with the SNAREs [15] , [21] , [23] , [50] or facilitating curvature of the presynaptic membrane [51] , [52] . Notably, recently an ~80% decrease in release has been demonstrated using a D229E mutation in Drosophila at the Ca 2+ -coordination site of C2A [53] , supporting the important function also of C2A in synchronous synaptic transmission. As a final remark, the membrane distance ruler developed in this study using membrane-anchored DNAs will also be very beneficial to the investigation of distance regulatory steps in other biological processes of interest, such as fertilization, viral entry as well as protein trafficking [54] , [55] , in which the gap between two membranes needs to be quantified at the nm-scale. Sample preparation Syt-1 (Rat) wild-type and the mutants were purified as previously described [28] and elaborated in Supplementary Methods . The DNA-lipid conjugates were synthesized by solid-phase synthesis using the lipid-phosphoramidite [26] as the last base under otherwise standard DNA synthesis conditions [56] and purified by RP-HPLC (see Supplementary Methods for details and characterization). Small unilammelar liposomes were prepared using Sephadex G-50 superfine (Sigma-Aldrich) size-exclusion columns. The size of the resulting liposomes was ~40 nm in diameter, estimated from the FCS information recorded simultaneously [57] and dynamic light scattering (DLS). Liposomes were labelled either with 0.5% OG-DHPE or with 1% TR-DHPE (Invitrogen), and the DNA/protein-to-lipid ratios were kept at 1:1,000. The proteoliposomes consisted of 20% DOPE, 10% cholesterol and 10% DOPS, whereas the acceptor liposomes contained 20% DOPE, 10% cholesterol, 15% DOPS and 2% PIP2, unless otherwise specified. Ten percent DOPS was included into all DNA liposomes. The remaining lipids were adjusted with DOPC to yield 100%. All non-labelled lipids were purchased from Avanti Polar Lipids. The buffer contained 150 mM KCl, 20 mM Hepes and was adjusted to pH 7.4. Hybridization of the DNA-liposomes was achieved by incubation for 5 min at 35 °C for 10 bp and 55 °C for 15 and 25 bp, followed by slow cooling back to room temperature. Syt-1 proteoliposomes were first incubated with the acceptor liposomes for 30 min and then added to buffers containing 1 mM EGTA or a final Ca 2+ concentration of 100 μM (checked with Fluo-5N, Invitrogen) for another 30 min to reach equilibrium. Final concentrations of donor liposomes were maintained at ~2 nM (one particle in the focal volume on average). Instrumentation Fluorescence microscopy measurements were performed on an Olympus IX71 inverted microscope with an UPlanSApo × 60/1.2 W water immersion objective. A Ti:sapphire oscillator (Chameleon, Coherent) centering at 800 nm served as the two-photon excitation source. A dichroic mirror 715DCSPXR (AHF) and a short pass filter E700SP were used to separate the excitation and emission and the dichroic mirror 590DCXR (AHF) to split the fluorescence onto the green and red avalanche photodiode detectors (SPCM-CD 2969, PerkinElmer), selected with band pass filters D525/20m and D680/30m (Chroma). Data were acquired with a router (PRT 400)-coupled TCSPC card (TimeHarp200, PicoQuant) and analysed with the SymPhoTime software version 5.3 (PicoQuant). Amplitude-weighted lifetime ( τ amp ) For numerical determination of the distances, we fitted all the fluorescence decay curves with iterative reconvolution using a model function of two exponential components: I ( t )= A 1 exp(− t / τ 1 )+ A 2 exp(− t / τ 2 ). The amplitude-weighted lifetime ( τ amp = a 1 τ 1 + a 2 τ 2 , where a 1 = A 1 /( A 1 + A 2 ) and a 2 = A 2 /( A 1 + A 2 )), which is more sensitive to changes in the faster component, was then calculated. How to cite this article: Lin, C.-C. et al. Control of membrane gaps by synaptotagmin-Ca 2+ measured with a novel membrane distance ruler. Nat. Commun. 5:5859 doi: 10.1038/ncomms6859 (2014).